Sumoylated hnRNPA2B1 controls the sorting of miRNAs into exosomes through binding to specific motifs Exosomes are released by most cells to the extracellular environment and are involved in cell-to-cell communication. Exosomes contain specific repertoires of mRNAs, microRNAs (miRNAs) and other non-coding RNAs that can be functionally transferred to recipient cells. However, the mechanisms that control the specific loading of RNA species into exosomes remain unknown. Here we describe sequence motifs present in miRNAs that control their localization into exosomes. The protein heterogeneous nuclear ribonucleoprotein A2B1 (hnRNPA2B1) specifically binds exosomal miRNAs through the recognition of these motifs and controls their loading into exosomes. Moreover, hnRNPA2B1 in exosomes is sumoylated, and sumoylation controls the binding of hnRNPA2B1 to miRNAs. The loading of miRNAs into exosomes can be modulated by mutagenesis of the identified motifs or changes in hnRNPA2B1 expression levels. These findings identify hnRNPA2B1 as a key player in miRNA sorting into exosomes and provide potential tools for the packaging of selected regulatory RNAs into exosomes and their use in biomedical applications. Exosomes are 50- to 300-nm-diameter vesicles secreted by most cells to the extracellular environment through fusion with the plasma membrane of endosomic compartments called multivesicular bodies [1] . Exosomes have been shown to contain RNAs, including mRNAs, microRNAs (miRNAs) and other non-coding RNAs [2] . These exosomes can be transferred to recipient cells, where shuttled RNA can be functional [3] , [4] , [5] , [6] , [7] . The functional relevance of miRNA-containing exosomes transfer has been reported both in vitro and in vivo [8] , [9] . Exosomes have potential uses as biomarkers [10] , [11] , vaccines [12] and vehicles for gene therapy [13] and have been modified to facilitate the delivery of cargo into specific target cells [14] . Recent evidence suggests that the miRNA repertoires of exosomes differ from those of their parental cells [5] , [15] , [16] ; however, the mechanisms that control the selective sorting of RNA into exosomes are still unknown. Here we identify short sequence motifs over-represented in miRNAs (EXOmotifs) that guide their loading into exosomes and show that their directed mutagenesis enables modulation of miRNA cargo in these vesicles. Heterogeneous nuclear ribonucleoprotein A2B1 (hnRNPA2B1) is a ubiquitously expressed RNA-binding protein that controls the transport and subcellular localization of specific mRNAs in neurons [17] and the trafficking of HIV genomic RNA [18] . We report that hnRNPA2B1 binds a specific subset of miRNAs through their EXOmotifs and controls their loading into exosomes. Moreover, hnRNPA2B1 in exosomes is sumoylated, and this post-translational modification controls hnRNPA2B1–miRNA binding. Specific repertoires of miRNAs are sorted into exosomes To assess whether some RNAs are specifically sorted into exosomes, we conducted a microarray analysis of activation-induced changes in the miRNA and mRNA profiles of primary T lymphoblasts and their exosomes ( Fig. 1a and Supplementary Data 1 , data publicly available at Gene Expression Omnibus through GEO Series accession number GSE50972 ). Exosome sample quality was assessed using western blot ( Supplementary Fig. S1a ) and electron microscopy ( Supplementary Fig. S1b ). Microarray analysis showed that in most cases the miRNAs modulated upon activation are not the same in cells and exosomes, either for upregulated or for downregulated miRNAs ( Fig. 1b , top panels). Thus, miRNAs whose expression levels increase in T cells upon activation are not significantly increased in exosomes and vice versa ( Supplementary Data 1 ). A similar trend was observed for mRNAs ( Supplementary Fig. S1c ). This lack of concordance between the activation-regulated miRNA and mRNA profiles of cells and exosomes indicates that miRNA and mRNA loading into exosomes is not a passive process. Several miRNAs were more highly represented in exosomes than in cells (such as miR-575, miR-451, miR-125a-3p, miR-198, miR-601 and miR-887; Fig. 1a ), and in most cases this difference is maintained under resting and activated conditions ( Fig. 1b , lower left panel). Similarly, most miRNAs that are more highly represented in cells than in exosomes (such as miR-17, mir-29a, let-7a, miR-142-3p, miR-181a and miR-18a; Fig. 1a ) maintain this tendency independently of the activation state of the cell ( Fig. 1b , lower right panel). Some miRNAs are thus specifically sorted into exosomes (EXOmiRNAs), whereas others are specifically retained in cells (CLmiRNAs). Similar results were obtained for mRNA ( Supplementary Fig. S1c ). Together, these data suggest the existence of mechanisms that control the active sorting of RNAs into exosomes. 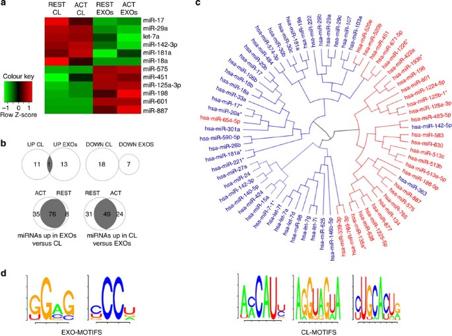Figure 1: The sequence of miRNAs controls their localization into exosomes. (a) Microarray analysis of exosomal and cellular miRNAs from human primary T lymphocytes in resting and activated (PMA and ionomycin) conditions. The panel shows the heatmap of the per-row normalized expression levels of selected miRNAs differentially expressed in cells (CL) versus exosomes (EXOs) in resting (REST) or activated conditions (ACT). (b) Upper panel: Venn diagrams based on miRNA microarray results showing that activation-induced changes in miRNA profile are not the same in T cells and their derived exosomes. Lower panel: Venn diagrams based on miRNA microarray results showing that some miRNAs are always specifically sorted into exosomes (EXOmiRNAs, left panel) or specifically retained in cells (CLmiRNAs, right panel), independently of the activation state of the T cell. (c) Cladogram showing the multiple alignment of mature sequences of 30 EXOmiRNAs (red) and 42 CLmiRNAs (blue), revealing that miRNA clustering coincides with preferential localization in exosomes or cells. (d) Over-represented motifs in EXOmiRNAs (EXOmotifs, left panels) and CLmiRNAs (CLmotifs, right panels); ZOOPS model was used. For each data set, the remaining miRNAs annotated in Ensembl was used as background. A Markov model of order 0 was assumed for the background sequences.E-value <10−4. Figure 1: The sequence of miRNAs controls their localization into exosomes. ( a ) Microarray analysis of exosomal and cellular miRNAs from human primary T lymphocytes in resting and activated (PMA and ionomycin) conditions. The panel shows the heatmap of the per-row normalized expression levels of selected miRNAs differentially expressed in cells (CL) versus exosomes (EXOs) in resting (REST) or activated conditions (ACT). ( b ) Upper panel: Venn diagrams based on miRNA microarray results showing that activation-induced changes in miRNA profile are not the same in T cells and their derived exosomes. Lower panel: Venn diagrams based on miRNA microarray results showing that some miRNAs are always specifically sorted into exosomes (EXOmiRNAs, left panel) or specifically retained in cells (CLmiRNAs, right panel), independently of the activation state of the T cell. ( c ) Cladogram showing the multiple alignment of mature sequences of 30 EXOmiRNAs (red) and 42 CLmiRNAs (blue), revealing that miRNA clustering coincides with preferential localization in exosomes or cells. ( d ) Over-represented motifs in EXOmiRNAs (EXOmotifs, left panels) and CLmiRNAs (CLmotifs, right panels); ZOOPS model was used. For each data set, the remaining miRNAs annotated in Ensembl was used as background. A Markov model of order 0 was assumed for the background sequences. E- value <10 −4 . Full size image miRNAs contain motifs that control their sorting in exosomes To investigate sequence differences, we performed a multiple alignment analysis (ClustalW) of the mature sequences of 30 EXOmiRNAs and 42 CLmiRNAs. For this analysis, we used EXOmiRNAs and CLmiRNAs that show differential expression in cells with respect to exosomes in both primary T cells (data from the current study) and the leukemic Jurkat T-cell line (data previously published in Mittelbrunn et al. [5] and publicly available at the Gene Expression Omnibus through GEO Series accession number GSE27997 ), and maintain this tendency under resting and activated conditions. The alignment cladogram grouped mature miRNAs according to their tendency to be localized in cells (CLmiRNAs, blue) or exosomes (EXOmiRNAs, red) ( Fig. 1c ). Moreover, paralogous miRNAs, which have similar sequences but differ in their chromosomal localization (and therefore in their transcription levels), always showed the same tendency to be localized in exosomes or cells ( Supplementary Data 1 ). In contrast, mature miRNA complementary chains derived from the same pre-miRNA, which are therefore expressed at similar levels but have different sequences, can differ in their tendency for cell versus exosome localization ( Supplementary Data 1 ). These data together suggest that the sequence of mature miRNAs is important for determining their sorting into exosomes. An unbiased search for specific motifs detected two motifs significantly over-represented in EXOmiRNAs (EXOmotifs), and three motifs significantly over-represented in CLmiRNA sequences (CLmotifs) ( Fig. 1d ). The EXOmotif GGAG and the CLmotif UGCA occur in the 3′ half of the miRNA sequence in 75% and 66.6% of cases, respectively. The other CLmotifs appear in the 5′ half, and the remaining EXOmotif does not occur at a characteristic position. To ascertain whether these motifs are important for miRNA sorting, we cloned the CLmiRNA miR-17 and the EXOmiRNA miR-601 into retroviral vectors and then performed directed mutagenesis to convert the CLmotif of miR-17 into an EXOmotif and, conversely, the EXOmotif of miR-601 into a CLmotif ( Fig. 2a ). Differential overexpression of wild-type versus mutated miRNAs was assessed using RT–PCR with locked nucleic acid (LNA)-specific primers, allowing us to discriminate between the wild-type and mutated miRNAs ( Supplementary Fig. S2 ). miRNA levels in Jurkat T cells and their exosomes were analysed by absolute quantitative PCR, normalizing against synthetic RNAs added exogenously to all samples. In accordance with microarray data ( Supplementary Table S1 ), the EXOmiRNAs miR-198 and miR-601 had a higher EXO/CL ratio than the CLmiRNAs miR-17 and miR-18a ( Fig. 2b ). However, conversion of the miR-17 CLmotif into an EXOmotif (miR-17mut) resulted in a higher EXO/CL ratio ( Fig. 2c , left panel), and in the complementary experiment conversion of the EXOmotif in miR-601 into a CLmotif (miR-601mut) decreased the EXO/CL ratio ( Fig. 2c , right panel). These data thus indicate that specific short motifs present in miRNAs determine the sorting of miRNAs into exosomes. 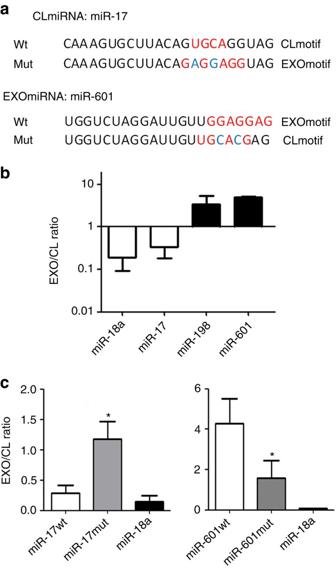Figure 2: Loading of miRNAs into exosomes is controlled by short motifs. (a) Sequences of wild-type miRNAs and their mutated versions used in this study. Mutated miR-17 has an EXOmotif instead of its characteristic CLmotif, whereas mutated miR-601 has a CLmotif instead of its EXOmotif. (b) EXO/CL ratio of each miRNA, obtained by dividing the number of copies in exosomes by the number of copies in cells. Copy number was determined using absolute quantitative PCR. Error bars represent s.d. (n=4). One-way ANOVA;P-value <0.01. (c) Left panel: EXO/CL ratio of mutated miR-17 and endogenous (wild-type) miR-17 and miR-18. Right panel: EXO/CL ratio of mutated miR-601 and endogenous (wild-type) miR-601 and miR-18a. Error bars represent s.d. (n=3). Student’st-test; *P-value <0.05. Figure 2: Loading of miRNAs into exosomes is controlled by short motifs. ( a ) Sequences of wild-type miRNAs and their mutated versions used in this study. Mutated miR-17 has an EXOmotif instead of its characteristic CLmotif, whereas mutated miR-601 has a CLmotif instead of its EXOmotif. ( b ) EXO/CL ratio of each miRNA, obtained by dividing the number of copies in exosomes by the number of copies in cells. Copy number was determined using absolute quantitative PCR. Error bars represent s.d. ( n =4). One-way ANOVA; P -value <0.01. ( c ) Left panel: EXO/CL ratio of mutated miR-17 and endogenous (wild-type) miR-17 and miR-18. Right panel: EXO/CL ratio of mutated miR-601 and endogenous (wild-type) miR-601 and miR-18a. Error bars represent s.d. ( n =3). Student’s t -test; * P -value <0.05. Full size image hnRNPA2B1 controls the loading of EXOmiRNAs into exosomes To investigate the molecular machinery that controls the sorting of specific miRNAs into exosomes, we screened for proteins present in exosomes that specifically bind EXOmiRNAs. Extracts from human primary T-cell exosomes were incubated with streptavidin beads coated with either a biotinylated EXOmiRNA (miR-198) or a biotinylated CLmiRNA (miR-17), and pulled down proteins were subjected to high-throughput identification using mass spectrometry ( Supplementary Data 2 ). As negative controls, we used non-coated and poly-A RNA-coated streptavidin beads. A group of RNA-related proteins was precipitated with one or both miRNAs, but not with the negative controls. Functional analysis of the precipitated proteins revealed a predominant association with biological functions related to RNA-post-transcriptional modifications ( Supplementary Table S1 ). The set of precipitated proteins included several heterogeneous nuclear ribonucleoproteins (hnRNPs). Among them, hnRNPA2B1 and hnRNPA1 seemed to bind only the EXOmiRNA, showing no detectable binding to CLmiRNA or the poly-A control ( Fig. 3 , Table 1 , Supplementary Fig. S3 and Supplementary Data 2 ). hnRNPA2B1 is an ubiquitous protein that has been shown to regulate mRNA trafficking to axons in neural cells [17] . Moreover, the mRNA transport function of hnRNPA2B1 in neurons is mediated by its binding to a 21-nt RNA sequence called RNA trafficking sequence (RTS) [19] . Interestingly, this sequence contains both of the EXOmotifs identified here ( Fig. 1d and Supplementary Fig. S4a ). HnRNPA2B1 is thus a good candidate regulator of EXOmiRNA sorting to exosomes. The presence of hnRNPA2B1 in exosomes was confirmed using western blot of exosomes isolated with ultracentrifugation and floated with centrifugation to equilibrium density into a sucrose gradient ( Supplementary Fig. S4b ). Although this is the most stringent method for exosome purification, we cannot rule out the presence of other extracellular vesicles with similar size and density in these fractions. Fluorescence-activated cell sorting (FACS) analysis showed that hnRNPA2B1 fluorescence is higher in permeabilized exosomes than in non-permeabilized exosomes ( Fig. 4a ), indicating that the protein locates inside the exosomes. Confocal analysis revealed that hnRNPA2B1 is located mainly in the nucleus, but also in cytoplasmic granules ( Supplementary Fig. S4c,d ). These data are supported using western blot analysis of hnRNPA2B1 in T-cell subcellular fractions, which show that hnRNPA2B1 cytoplasmic fraction is mainly associated with membranous organelles ( Supplementary Fig. S4e ). Moreover, hnRNPA2B1 colocalizes in the cytoplasm of cells with MVB markers such as ceramide [20] ( Supplementary Fig S5 ). 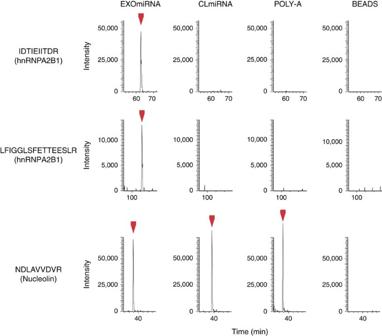Figure 3: HnRNPA2B1 specifically binds EXOmiRNAs. Exosome extracts were incubated with streptavidin beads coated with either a biotinylated EXOmiRNA (miR-198), a biotinylated CLmiRNA (miR-17) or a negative control (poly-A), and with non-coated beads (beads). The graphs represent the extracted ion chromatogram traces of the monoisotopic peaks corresponding to the indicated peptides, identified from hnRNPA2B1or from a non-specifically binding protein (nucleolin). Figure 3: HnRNPA2B1 specifically binds EXOmiRNAs. Exosome extracts were incubated with streptavidin beads coated with either a biotinylated EXOmiRNA (miR-198), a biotinylated CLmiRNA (miR-17) or a negative control (poly-A), and with non-coated beads (beads). The graphs represent the extracted ion chromatogram traces of the monoisotopic peaks corresponding to the indicated peptides, identified from hnRNPA2B1or from a non-specifically binding protein (nucleolin). Full size image Table 1 Summary of high-throughput mass spectrometry analysis of miRNA-precipitated proteins. 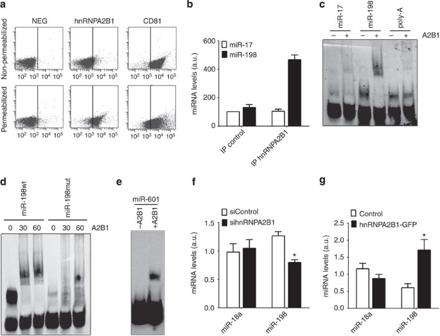Figure 4: HnRNPA2B1 binds EXOmiRNAs through EXOmotifs and is involved in their loading into exosomes. (a) FACS analysis of hnRNPA2B1 and CD81 in exosome-coupled beads. Exosomes were coupled to aldehyde-sulfate beads, permeabilized or left intact and incubated with antibodies to hnRNPA2B1 (middle panels) or CD81 (right panels) and secondary antibody. Exosome-coupled beads incubated with secondary antibody alone were used as negative controls (left panels). (b) qPCR analysis of miRNAs contained in hnRNPA2B1 immunoprecipitates from exosome lysates, showing the specific binding of miR-198 to hnRNPA2B1 in exosomes. Immunoprecipitation was performed with magnetic beads coated with anti-hnRNPA2B1 or anti-IgG1 control antibody. Data are presented relative to miR-17 content in control immunoprecipitates. Error bars represent s.d. (n=2). (c) Electrophoresis mobility shift assay showing the specific binding of miR-198 to hnRNPA2B1. Biotinylated miR-17, miR-198 or poly-A were incubated with or without purified human hnRNPA2B1 as indicated. (d) Electrophoresis mobility shift assay showing the binding of hnRNPA2B1 to wild-type and mutated miR-198. Biotinylated wild-type and mutated miR-198 were incubated with or without purified human hnRNPA2B1 as indicated. Numbers represent protein concentration (ng μl−1). (e) Electrophoresis mobility shift assay showing the binding of hnRNPA2B1 to miR-601. (f) qPCR analysis of miR-18a and miR-198 in exosomes from control cells or cells silenced with siRNAs against hnRNPA2B1. Bars represent miRNA levels in exosomes (arbitrary units). Error bars represent s.d. (n=3). Student’st-test; *P-value <0.001. (g) qPCR analysis of miR-18a and miR-198 levels in exosomes from control cells or cells overexpressing hnRNPA2B1-GFP. Bars represent miRNA levels in exosomes (arbitrary units). Error bars represent s.d. (n=3). Student’st-test; *P-value<0.01. Full size table Figure 4: HnRNPA2B1 binds EXOmiRNAs through EXOmotifs and is involved in their loading into exosomes. ( a ) FACS analysis of hnRNPA2B1 and CD81 in exosome-coupled beads. Exosomes were coupled to aldehyde-sulfate beads, permeabilized or left intact and incubated with antibodies to hnRNPA2B1 (middle panels) or CD81 (right panels) and secondary antibody. Exosome-coupled beads incubated with secondary antibody alone were used as negative controls (left panels). ( b ) qPCR analysis of miRNAs contained in hnRNPA2B1 immunoprecipitates from exosome lysates, showing the specific binding of miR-198 to hnRNPA2B1 in exosomes. Immunoprecipitation was performed with magnetic beads coated with anti-hnRNPA2B1 or anti-IgG1 control antibody. Data are presented relative to miR-17 content in control immunoprecipitates. Error bars represent s.d. ( n =2). ( c ) Electrophoresis mobility shift assay showing the specific binding of miR-198 to hnRNPA2B1. Biotinylated miR-17, miR-198 or poly-A were incubated with or without purified human hnRNPA2B1 as indicated. ( d ) Electrophoresis mobility shift assay showing the binding of hnRNPA2B1 to wild-type and mutated miR-198. Biotinylated wild-type and mutated miR-198 were incubated with or without purified human hnRNPA2B1 as indicated. Numbers represent protein concentration (ng μl −1 ). ( e ) Electrophoresis mobility shift assay showing the binding of hnRNPA2B1 to miR-601. ( f ) qPCR analysis of miR-18a and miR-198 in exosomes from control cells or cells silenced with siRNAs against hnRNPA2B1. Bars represent miRNA levels in exosomes (arbitrary units). Error bars represent s.d. ( n =3). Student’s t -test; * P -value <0.001. ( g ) qPCR analysis of miR-18a and miR-198 levels in exosomes from control cells or cells overexpressing hnRNPA2B1-GFP. Bars represent miRNA levels in exosomes (arbitrary units). Error bars represent s.d. ( n =3). Student’s t -test; * P -value<0.01. Full size image Specific binding of hnRNPA2B1 to miR-198 was verified with immunoprecipitation of hnRNPA2B1 from exosome lysates followed by qPCR of miRNAs; miR-198, but not miR-17, was amplified from hnRNPA2B1 immunoprecipitates, demonstrating specific binding of hnRNPA2B1 and miR-198 in exosomes in vivo ( Fig. 4b ). The specific binding of hnRNPA2B1 and miR-198 was confirmed using electrophoresis mobility shift assay ( Fig. 4c ). This binding was inhibited when the EXOmotif of miR-198 was mutated ( Fig. 4d ), indicating that the binding of hnRNPA2B1 to miR-198 is dependent on the presence of the EXOmotif. HnRNPA2B1 also binds other EXOmiRNAs such as miR-601 ( Fig. 4e ). In order to investigate the role of hnRNPA2B1 in the packaging of miRNAs into exosomes, we assessed the effect of silencing or increasing its expression on the EXO miRNA profile in Jurkat T cells ( Supplementary Fig. S6a,b ). HnRNPA2B1 silencing significantly decreased the levels of the EXOmiRNA miR-198 in exosomes but did not significantly alter the levels of the CLmiRNA miR-18a ( Fig. 4f ); in contrast, hnRNPA2B1 overexpression increased the levels of miR-198 in exosomes without changing the levels of miR-18a ( Fig. 4g ). In the overexpression experiments, the purification method used to recover exosomes was less stringent; therefore, it is possible that we were also detecting exosome-independent secreted miRNAs. These data indicate that hnRNPA2B1 controls the loading of specific EXOmiRNAs into exosomes. The loading of miRNAs is controlled by hnRNPA2B1 sumoylation Western blot analysis of hnRNPA2B1 ( Fig. 5a ) and hnRNPA1 ( Supplementary Fig. S7a ) from exosomes revealed a higher molecular weight (m.w.) (~10–12 kDa more) in comparison with cells, suggesting that these proteins might be post-translationally modified in exosomes. Several hnRNPs including hnRNPA1 are known to attach to small ubiquitin-related modifier (SUMO) [21] , and the observed m.w. changes in exosomes are consistent with sumoylation. Moreover, in silico analysis of the hnRNPA2B1 protein sequence identified several predicted sites for SUMO conjugation ( Supplementary Fig. S7b ). To assess hnRNPA2B1 sumoylation, HEK293T cells were co-transfected with SUMO-1 and hnRNPA2B1-GFP (green-fluorescent protein) or GFP plasmids. After GFP immunoprecipitation, SUMO-1 was detected in cells transfected with hnRNPA2B1GFP but not in cells transfected with GFP alone ( Fig. 5b ). Sumoylation of hnRNPA2B1 was also demonstrated in T cells by the detection of SUMO-1 after hnRNPA2B1 immunoprecipitation ( Fig. 5c ). To confirm whether the higher m.w. of exosomal hnRNPA2B1 was because of sumoylation, we cultured Jurkat T cells in the presence of the specific sumoylation inhibitor anacardic acid (AA) [22] ( Supplementary Fig. S7c ). Whereas untreated exosomes contained barely detectable amounts of low-m.w. hnRNPA2B1, in the presence of AA the low-m.w. band could be readily detected ( Fig. 5d ). These results indicate that the higher m.w. of exosomal hnRNPA2B1 is because of sumoylation, and that sumoylated hnRNPA2B1 is preferably sorted to exosomes. Further analysis revealed that treatment with AA reduced the levels of miR-198 in exosomes, whereas the levels of miR-17 and miR-18 did not change ( Fig. 5e ). Moreover, hnRNPA2B1 IP-qPCR experiments showed that there was less miR-198 bound to hnRNPA2B1 when sumoylation was inhibited ( Fig. 5f ), while exosome secretion or cell death did not change ( Supplementary Fig. S7d ). These data indicate that hnRNPA2B1-mediated loading of EXOmiRNAs into exosomes is controlled by the sumoylation of the protein. 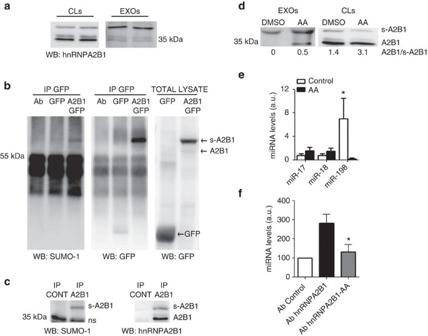Figure 5: hnRNPA2B1 is sumoylated in exosomes and this modification controls its binding to miRNAs. (a) Representative western blot analysis showing hnRNPA2B1 in T cells and their exosomes. (b) Western blot analysis of hnRNPA2B1 sumoylation. HEK293T cells were co-transfected with SUMO-1 and hnRNPA2B1-GFP or GFP plasmids. GFP immunoprecipitates and total lysates were immunoblotted for SUMO-1 and/or GFP. Ab: antibody-conjugated Dynabeads without cell lysates. GFP: lysates from cells transfected with GFP and SUMO-1. hnRNPA2B1-GFP: lysates from cells transfected with hnRNPA2B1-GFP and SUMO-1. (c) Western blot analysis of hnRNPA2B1 sumoylation in T cells. hnRNPA2B1 was immunoprecipitated from Jurkat T cells and immunoblotted for SUMO-1 and hnRNPA2B1. A2B1: hnRNPA2B1; s-A2B1: sumoylated hnRNPA2B1; ns: nonspecific band. IP CONT: immunoprecipitation with control antibody. IP A2B1: immunoprecipitation with hnRNPA2B1 antibody. (d) Western blot analysis of hnRNPA2B1 molecular weight in exosomes and cells in the presence of the sumoylation inhibitor AA or vehicle (DMSO). Numbers below the lanes are the densitometry ratios of total hnRNPA2B1 to sumoylated hnRNPA2B1. (e) qPCR analysis of miRNA levels in exosomes from control or AA-treated cells. Bars represent miR-17, miR-18 and miR-198 levels (arbitrary units). Error bars represent s.d. (n=3). Students’sttest; *P-value <0.05. (f) qPCR analysis of miR-198 in hnRNPA2B1 immunoprecipitates from exosome lysates derived from control or AA-treated cells, showing decreased binding of miR-198 to hnRNPA2B1 in the presence of AA. Bars represent miR-198 levels (arbitrary units). Data are presented relative to the control condition. Error bars represent s.d. (n=3). Student’st-test; *P-value<0.05. Figure 5: hnRNPA2B1 is sumoylated in exosomes and this modification controls its binding to miRNAs. ( a ) Representative western blot analysis showing hnRNPA2B1 in T cells and their exosomes. ( b ) Western blot analysis of hnRNPA2B1 sumoylation. HEK293T cells were co-transfected with SUMO-1 and hnRNPA2B1-GFP or GFP plasmids. GFP immunoprecipitates and total lysates were immunoblotted for SUMO-1 and/or GFP. Ab: antibody-conjugated Dynabeads without cell lysates. GFP: lysates from cells transfected with GFP and SUMO-1. hnRNPA2B1-GFP: lysates from cells transfected with hnRNPA2B1-GFP and SUMO-1. ( c ) Western blot analysis of hnRNPA2B1 sumoylation in T cells. hnRNPA2B1 was immunoprecipitated from Jurkat T cells and immunoblotted for SUMO-1 and hnRNPA2B1. A2B1: hnRNPA2B1; s-A2B1: sumoylated hnRNPA2B1; ns: nonspecific band. IP CONT: immunoprecipitation with control antibody. IP A2B1: immunoprecipitation with hnRNPA2B1 antibody. ( d ) Western blot analysis of hnRNPA2B1 molecular weight in exosomes and cells in the presence of the sumoylation inhibitor AA or vehicle (DMSO). Numbers below the lanes are the densitometry ratios of total hnRNPA2B1 to sumoylated hnRNPA2B1. ( e ) qPCR analysis of miRNA levels in exosomes from control or AA-treated cells. Bars represent miR-17, miR-18 and miR-198 levels (arbitrary units). Error bars represent s.d. ( n =3). Students’s t test; * P -value <0.05. ( f ) qPCR analysis of miR-198 in hnRNPA2B1 immunoprecipitates from exosome lysates derived from control or AA-treated cells, showing decreased binding of miR-198 to hnRNPA2B1 in the presence of AA. Bars represent miR-198 levels (arbitrary units). Data are presented relative to the control condition. Error bars represent s.d. ( n =3). Student’s t -test; * P -value<0.05. Full size image In this report we identify short sequence motifs over-represented in miRNAs commonly enriched in exosomes. These motifs control the loading of these miRNAs into exosomes, and their directed mutagenesis enables the modulation of miRNA cargo in these vesicles. The ability of short nucleotide sequences to guide the transport of RNAs to different subcellular compartments has been reported previously. For example, a 20-ribonucleotide stem-loop sequence was shown to direct the import of nuclear-encoded mRNAs to mitochondria [23] , and the hexanucleotide terminal motif of miR-29b was previously demonstrated to direct the nuclear enrichment of this miRNA [24] . In addition, a 21-nucleotide sequence in the 3′ untranslated region (UTR) of the myelin basic protein (MBP) mRNA was demonstrated to be necessary and sufficient for the transport of this transcript along axons and its subsequent localization in the myelin compartment [25] . This sequence, known as RTS, binds the protein hnRNPA2B1, which is required for MBP transport and localization [17] , [19] . Our proteomic analyses detected the specific binding of hnRNPA2B1 to the EXOmiRNA miR-198, which shares with the RTS the two motifs we found to be over-represented in EXOmiRNAs. We have demonstrated that hnRNPA2B1, which is present in exosomes, binds the EXOmiRNA directly and controls its loading into these microvesicles. In addition, hnRNPA2B1 in exosomes is preferentially sumoylated, and this sumoylation is important for the loading of EXOmiRNAs into exosomes. HnRNPA1 might work in a similar way, since it specifically binds the EXOmiRNA miR-198 and has been reported to be sumoylated [21] . Interestingly, hnRNPA1 has been implicated in miRNA biogenesis [26] . Unlike ubiquitination, sumoylation does not target proteins to proteasome degradation; instead, conjugation of SUMO has been shown to affect protein functions by altering their stability, subcellular localization or their ability to interact with other proteins [27] . Interestingly, modification of protein properties by sumoylation has been reported to affect mRNA trafficking in axons by promoting the binding of the La protein to dynein over the binding to kinesin [28] . SUMO conjugation has been demonstrated to affect several hnRNPs [21] , whose functions can also be modified by other post-translational modifications such as phosphorylation. In this regard, the interaction of hnRNPA2B1 and hnRNPF with MBP mRNA can be modulated through phosphorylation by src-kinases [29] , [30] . Moreover, sumoylation and phosphorylation are associated events in many pathways; for instance, FAK protein sumoylation enables its interaction with src-kinases, resulting in phosphorylation and full activation of the protein [31] . The function of hnRNPA2B1 in transporting RNA to exosomes is probably dependent on its ability to interact with cytoskeletal components. Indeed, there is evidence that in neurons hnRNPA2B1 partly regulates motor activity through indirect contacts with microtubules [32] , and monomeric or short oligomeric actin has been shown to associate with a subset of hnRNPs, including hnRNPA2B1 [33] . HnRNPA2B1 was demonstrated to control HIV RNA trafficking and viral assembly [18] , and given the convergences between HIV virus production and exosome biogenesis and secretion [34] , [35] , it is conceivable that both phenomena share common RNA transport mechanisms. In addition, hnRNPA2B1 and hnRNPA1 contain prion-like domains [36] that correspond to the ‘low-complexity sequences’ found in several hnRNPs that are essential determinants of RNA granule assembly [37] . Prion-like domains are also involved in hnRNPA2B1 recruitment to stress granules [36] , which are cytoplasmatic ribonucleoprotein granules containing nontranslated mRNA and translation repressors [38] . Finally, hnRNPA2B1 has also been described to interact with TDP-43 (ref. 39 ), another component of RNP granules that has been implicated in miRNA biogenesis [40] . Certain conserved RNA motifs are commonly present in specific secondary structures called RNA tetraloops, which usually serve as recognition sites for interaction with proteins or other RNA structural elements. The GGAG tetraloop has been reported to mediate the binding of HIV nucleocapsid protein to genomic ψRNA packaging signals [41] , and also mediates RNA–protein interactions in the signal recognition particle complex [42] . It would be interesting to study whether the GGAG EXOmotif occurs in specific secondary structures in EXO miRNAs and whether these putative structures are essential for the binding to hnRNPA2B1. Cells have recently been shown to communicate with each other through the transfer of miRNA-loaded exosomes [5] , [6] , [7] , [8] , [9] . For example, monocyte-derived exosomes deliver miR-150 to endothelial cells and enhance their migration by reducing c-myb expression [9] . The miRNA content of exosomes plays a critical role in this type of cell–cell communication and determines the fate of the recipient cell. Thus, exosomes derived from the bone marrow mesenchymal stromal cells of myeloma patients promote tumour growth, and this effect depends on the content of miR-15a in exosomes [8] . HnRNPA2B1-mediated miRNA loading into exosomes is probably important for this novel mode of cell–cell communication. However, the functional relevance of hnRNPA2B1 and how it is regulated in different cell situations is still not understood. Another possible function for hnRNPA2B1-dependent export of miRNAs in exosomes is to provide a mechanism for eliminating undesired miRNAs. Our findings show that sumoylated hnRNPA2B1 directs the loading of certain miRNAs into exosomes through recognition of specific short motifs ( Fig. 6 ). These RNA motifs may be useful for the artificial loading of selected small regulatory RNAs into exosomes and may prove to be suitable tools for the engineering of exosomes for gene therapy. These findings represent a major advance in our understanding of how miRNAs are loaded into exosomes and exported from cells. 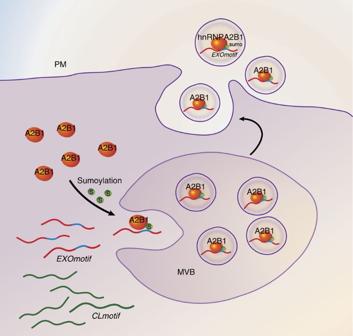Figure 6: Diagram representing the proposed mechanism of the sorting of miRNA into exosomes through binding to hnRNPA2B1. PM: plasma membrane, MVB: multivesicular bodies, S: SUMO, A2B1: hnRNPA2B1. Figure 6: Diagram representing the proposed mechanism of the sorting of miRNA into exosomes through binding to hnRNPA2B1. PM: plasma membrane, MVB: multivesicular bodies, S: SUMO, A2B1: hnRNPA2B1. Full size image Cell culture Human peripheral blood mononuclear cells were isolated from buffy coats from healthy donors by separation on a biocoll gradient (Biochrom). After 30 min of adhesion step at 37 °C, non-adherent cells were cultured 2 days in the presence of phytohemagglutinin (5 μg ml −1 ) to induce lymphocyte proliferation. To obtain T lymphoblasts, IL-2 (50 U ml −1 ) was added to the medium every 2 days for a time period of 5 days. When indicated, T lymphoblasts were activated with phorbol myristate acetate (PMA) (50 ng ml −1 ) plus ionomycin (500 ng ml −1 ). The human Jurkat-derived T-cell line J77cl20 (TCR Vαl. 2 Vβ8) was cultured in RPMI (Sigma) containing 10% fetal bovine serum (FBS; Invitrogen). Jurkat cells were transduced by retroviral infection to overexpress miR-17mut or miR-601mut and selected with puromycin (4 μg ml −1 ). HEK-293T cells were cultured in DMEM (Sigma) containing 10% FBS. All the procedures and techniques developed within this work have been performed with the approval of the Ethical Committee from Centro Nacional de Investigaciones Cardiovasculares Carlos III, with the required ethical authorization and following both Spanish and the European Union rules and laws. Exosome purification Donor cells were cultured in RPMI-1640 supplemented with 10% FBS (depleted of bovine exosomes by overnight centrifugation at 100,000 g ). Exosomes were prepared from cell supernatants by a series of centrifugation and filtration steps [3] ; briefly, cells were centrifuged (320 g , 5 min) and the supernatant filtered through 0.22-μm membranes. Exosomes were pelleted using ultracentrifugation at 100,000 g for 60 min at 4 °C (Optima L-100 XP, Beckman Coulter). When indicated, exosomes were overlaid with a linear sucrose gradient (2.5–0.4 M sucrose in phosphate-buffered saline (PBS)) and floated into the gradient using centrifugation for 16 h at 120,000 g . For the analysis of miRNA profile in cells overexpressing hnRNPA2B1, exosomes were isolated with ExoQuick-TC Exosome Precipitation Solution (SBI). Microarray analysis Primary human T lymphoblasts were obtained from eight donors and total RNA was isolated from cells and derived exosomes before and after activation with PMA (50 ng ml −1 ) plus ionomycin (500 ng ml −1 ). Cell activation was assessed using flow cytometry analysis of CD69 upregulation. The large and small RNA profiles of cells and exosomes were assessed on an Agilent 2100 Bioanalyzer (Agilent) by analysis of total RNA (RNA nano chips) and small RNA (small RNA chips). Microarray experiments were performed using the human miRNA and mRNA microarrays from Agilent. Arrays were used to analyse two RNA pools from four healthy donors of primary human resting and activated T lymphoblasts and their exosomes. Array data for mRNA and miRNA were normalized using the quantiles method (similar results were obtained for miRNA data using vsn2 normalization). After normalization, only those miRNA probes present in at least two samples and with an average expression above the 20th percentile of all average expressions were considered for further analysis (316 miRNAs). Similarly, probes from genes included in the mRNA array were excluded from the analysis unless they exhibited a strong signal and an acceptable flag in all replicates of at least one studied condition, and these probes were additionally required to present some changes across samples (CV >5%). Linear models [43] as implemented in the limma Bioconductor package were then used to find miRNAs and genes differentially expressed between the contrasts of interest. We considered differentially expressed those mRNAs and miRNAs with an adjp ≤0.05. Multiple alignment and over-represented motif analysis Multiple sequence alignment was performed with ClustalW (gap open 12, gap extension 3). The cladogram was generated with the Geneious software. An unbiased search to identify over-represented motifs was performed using the bioconductor package COSMO [44] . COSMO results were replicated using Improbizer. We ran the ZOOPS (zero-or-one-occurrence) model to find over-represented 4–8 nucleotide-long motifs. For each data set, the remaining miRNAs annotated in Ensembl was used as background. A Markov model of order 0 was assumed for the background sequences. All motifs showed an E -value <10 −4 . Cloning and directed mutagenesis hsa-miR-17 (forward primer: 5′-CCCTTTCTCGAGCCCCATTAGGGATTATGCTG-3′, reverse primer: 5′-GGGAAAGAATTCAGATGCACCTTAGAACAAAAAGC-3′) and hsa-miR-601 (forward primer: 5′-CCCTTTCTCGAGGAGCACAGCCCTCAGTCTCT-3′, reverse primer: 5′-GGGAAAGAATTCTCCAACTCTGACTGGGACCT-3′) were cloned in pGEM-T (Promega) and subsequently in pLVX-AcGFP1-C1 (miR-17) or pMSCV-GFP (miR-601) in Xho I and Eco RI restriction sites. Site-directed mutagenesis was performed with the QuickChange Site-Directed mutagenesis kit (Stratagene). Constructs were sequence-verified. Lentiviral infection Jurkat cells overexpressing miRNA-17mut or miRNA-601mut were generated by retroviral infection. Briefly, HEK293T cells were co-transfected (Lipofectamine 2000, Invitrogen) with plasmids encoding the desired miRNA and pCL-Ampho plasmid (RetroMax). Supernatants were collected after 48 h, filtered (0.45 μm) and added to Jurkat T cells. Cells were centrifuged (1,200 g , 2 h) and incubated for 6 h at 37 °C. Medium was replaced with RPMI, and GFP-expressing cells were selected using flow cytometry sorting. RNA isolation Total RNA was extracted with QIAzollysis reagent (Qiagen) and the miRNeasy mini kit (Qiagen) and was screened for purity and concentration in a Nanodrop-1000 Spectrophotometer (Thermo Scientific). RNA integrity was assessed by ethidium bromide labeling on a 1.5% agarose gel. Reverse transcription and quantitative real-time PCR cDNA was synthesized and mature miRNAs were quantified with miRCURY LNA Universal RT microRNA PCR (Exiqon), using miRNA LNA primers (Exiqon) and SYBRgreen PCR master mix (Applied Biosystems). PCR reactions were performed in triplicate in 10 μl volumes in 384-well plates. Quantitative miRNA expression data were acquired and analysed using the ABI Prism 7900HT Sequence Detection System (Applied Biosystems). Data were further analysed using BiogazelleQBasePlus software (Biogazelle). In relative PCR quantifications, RNU1A1 and RNU5G were used as endogenous controls and results are expressed in arbitrary units. In absolute PCR quantifications 10-fold dilutions of synthetic RNA oligonucleotides (Exiqon) at known concentrations were reverse-transcribed and amplified, and the absolute amount of each miRNA was calculated from the standard curve. A total of 10 8 copies of synthetic spike-in RNA (Exiqon) were also added to each sample for normalization between samples. EXO/CL ratios were calculated by dividing the number of copies in exosomes by the number of copies in cells. Overexpression Jurkat cells were transfected with hnRNPA2B1-GFP (Origene) by electroporation. Cells were resuspended in Opti-MEM (GIBCO; 5 × 10 7 cells per ml) with 30 μg of DNA plasmid and electroporated with Gene PulserXcell (Bio-Rad) at 1,200 μFa, 240 mV for 30 ms in 4 mm Bio-Rad cuvettes (Bio-Rad), and hnRNPA2B1-GFP-positive cells were FACS-sorted. HEK 293T cells were co-transfected with SUMO-1-HIS (kindly provided by Dr G. Bossis, IGMM Montpellier) and hnRNPA2B1-GFP (Origene) or GFP-turbo by Lipofectamine-2000 (Invitrogen) according to the manufacturer’s instructions. Silencing Jurkat cells were transfected twice (48 h apart) with a pool of double-stranded siRNAs targeting hnRNPA2B1 (forward 5′-GCAAGACCUCAUUCAAUUGUU-3′, reverse 5′-CCAUUGAAUGAGGUCUUGCUU-3′; forward 5′-GAACAAUGGGGAAAGCUUAUU-3′, reverse 5′-UAAGCUUUCCCCAUUGUUCUU-3′; forward 5′-GUUCAGAGUUCUAGGAGUCUU-3′, reverse 5′-CACUCCUAGAACUCUGAACUU-3′; forward 5′-GAAGAGUAGUUGAGCCAAAUU-3′, reverse 5′-UUUGGCUCAACUACUCUUCUU-3′) (Eurogentec). Control cells were transfected with a control siRNA (forward 5′-AAUUCUCCGAACGUGUCACGUUU-3′, reverse 5′-ACGUGACACGUUCGGAGAAUUUU-3′) (Eurogentec). Cells were resuspended in Opti-MEM (GIBCO; 5 × 10 7 cells per ml) with 2 μM siRNA and electroporated with Gene PulserXcell (Bio-Rad) at 240 mV for 28 ms in 4 mm Bio-Rad cuvettes (Bio-Rad). Flow cytometry analysis and sorting Cell samples were analysed with a FACSCanto flow cytometer and FACSDiva software (BD Biosciences). Viable cells were identified by propidium iodide exclusion. Cells were sorted on a FACSAria flow cytometer (BD Biosciences). miRNA pull-down Exosomes from human primary T cells were isolated, resuspended in 400 μl buffer 1 and precleared by incubation with streptavidin–sepharose beads (GE Healthcare) (1.5 h, 4 °C). Biotinylated miRNAs or poly-A (20 nmol; Dharmacon) were resuspended in TBS with RNAse inhibitor (40 U ml −1 ; Invitrogen) and incubated with 40 μl streptavidin–sepharose beads (4 h, 4 °C). Beads were washed twice with TBS and incubated with lysates (O/N, 4 °C). Beads were washed six times in buffer 2. Protein loading buffer (Fermentas) was added and beads were heated at 90° for 10 min before proteomics analysis. See Supplementary Methods for buffer compositions. Protein identification using mass spectrometry Proteins were in-gel digested using a previously described protocol [45] . Briefly, 75 μl of beads were suspended in 25 μl sample buffer and loaded in 2.8-cm-wide wells of an SDS–PAGE gel. The run was stopped as soon as the front entered 3 mm into the resolving gel; the protein band was visualized with Coomassie staining, excised and digested overnight at 37 °C with 60 ng μl −1 trypsin at 5:1 protein:trypsin (w/w) ratio in 50 mM ammonium bicarbonate, pH 8.8 containing 10% acetonitrile. The resulting tryptic peptides were extracted by 1 h incubation in 12 mM ammonium bicarbonate, pH 8.8. TFA was added to a final concentration of 1% and the peptides were finally desalted on C18 Oasis cartridges and dried down. Peptide identification using mass spectrometry was performed as described [46] . Briefly, the peptides were resuspended and injected on a C-18 reversed phase nano-column (75 μm I.D. × 25 cm, Acclaim PepMap100, Thermo Scientific) and analysed in a continuous acetonitrile gradient consisting of 0–43% B in 90 min, 50–90% B in 1 min (B=90% acetonitrile, 0.5% acetic acid). A flow rate of ca. 300 nl min −1 was used to elute peptides from the reversed phase nanocolumn to an emitter nanospray needle for real time ionization and peptide fragmentation on an LTQ XP Orbitrap mass spectrometer (Thermo Fisher). An enhanced FT spectrum (30.000 resolution) followed by MS/MS spectra from most intense 10 parent ions were performed along the chromatographic run (130 min). Dynamic exclusion was set at 30 s. The MS/MS raw files were searched against the Human Swissprot database (Uniprot release 14.0, 19929 sequence entries for human) supplemented with porcine trypsin and bacterial Streptavidin. SEQUEST results were validated using the probability ratio method [47] and false discovery rates were calculated using the refined method [48] . Peptide and scan-counting was performed assuming as positive events those with a FDR equal to or lower than 5%. Immunoprecipitation A total of 3 × 10 7 cells were lysed in 1 ml of buffer 4 and incubated for pre-clearing with pre-washed Protein G Dynabeads (Invitrogen) (50 μl per condition) (1 h, 4 °C). A total of 50 μl of Dynabeads were washed twice in buffer 3, and resuspended in 200 μl of buffer 3 containing 10 μg mouse anti-hnRNPA2B1 (Santa Cruz), rabbit anti-GFP-turbo (Pierce), or mouse anti-IgG control (Santa Cruz), and incubated 1 h at room temperature. Pre-cleared lysates were incubated with Ab-conjugated Dynabeads (1.5 h, 4 °C). Ab-conjugated Dynabeads were washed twice with buffer 4, three times with buffer 5, transferred to clean tubes and washed with buffer 6. Protein Loading buffer (Fermentas) was added, samples were boiled at 95 °C for 5 min and processed for immunoblotting. Immunoblotting Cells or exosomes were lysed in lysis buffer (25 mM Tris pH8, 150 mM NaCl, 2 mM MgCl 2 , 0.5%NP-40,) containing a protease inhibitor cocktail (Complete, Roche). Proteins were separated on 10% acrylamide/bisacrylamide gels and transferred to a nitrocellulose membrane. Membranes were incubated with specific primary antibodies (5 μg ml −1 ) and peroxidase-conjugated secondary antibodies (5 μg ml −1 ), and proteins were visualized with LAS-3000. The following antibodies were used: mouse anti-hnRNPA1 (R4528, Sigma) (1:1,000), mouse anti-hnRNPA2B1 (sc-53531, Santa Cruz) (1:200), goat anti-SUMO1 (sc-6376, Santa Cruz) (1:200), mouse anti-SUMO1 (ab93951, Abcam) (1:1,000), goat anti-mouse peroxidase (31446, Thermo Scientific) (1:5,000) and goat anti-rabbit peroxidase (37460, Thermo Scientific) (1:5,000). Band intensities were quantified with Image Gauge. Full blots are shown in Supplementary Fig. S8 . Immunoprecipitation–qPCR Protein G Dynabeads (50 μl per condition) (Invitrogen) were washed twice in buffer 3 and resuspended in 200 μl of buffer 3 containing 10 μg mouse anti-hnRNPA2B1 (Santa Cruz) or mouse anti-IgG control (Santa Cruz) and incubated overnight at 4 °C. Exosomes were isolated, resuspended in cold PBS and UV-crosslinked (120 mJ cm −2 at 254 nm) (Stratalinker UV crosslinker, Stratagene). Crosslinked exosomes were ultracentrifugated, lysed by resuspension in buffer 4 and incubated (1 h, 4 °C) with non-conjugated Dynabeads (50 μl per condition). The precleared lysates were incubated with 50 μl of Ab-conjugated Dynabeads (1.5 h, 4 °C), which were then washed twice with buffer 4 and three times with buffer 5, and transferred to clean tubes and washed with buffer 6. For protein detection, Protein Loading buffer (Fermentas) was added, and samples were boiled at 70 °C for 10 min and processed for immunoblotting. For qPCR analysis, 700 μl of Qiazol lysis reagent (Qiagen) were added and samples were vortexed. See Supplementary Methods for buffer compositions. Electrophoresis mobility shift assay Biotinylated miRNAs or poly-A (1 nmol) (Dharmacon) were incubated (when indicated) with 3 μg purified human hnRNPA2B1 protein (Origene) in electrophoresis mobility shift assay (EMSA) buffer (20 min at room temperature). EMSA was performed with the Light Shift Chemiluminescent EMSA kit (Pierce). FACS analysis of exosome-coupled beads Exosomes were obtained using ultracentrifugation and sucrose gradient flotation, resuspended in PBS and coupled to 4 μm aldehyde-sulfate beads (Invitrogen) overnight at room temperature in rotation. Beads were washed and blocked for 60 min at room temperature in 4% bovine serum albumin in PBS. For intracellular staining, bead-bound exosomes were permeabilized and fixed for 5 min at room temperature with 0.2% Triton X-100, 2% formaldehyde in PBS. Beads were incubated with anti-hnRNPA2B1 (Santa Cruz) or anti-CD81 (5A6, Santa Cruz) for 1 h at 4 °C, washed and incubated with Alexa-488-goat-anti-mouse IgG (Invitrogen) for 30 min. Beads were acquired on a FACSCalibur (BD) and data were analysed with FlowJo software (Tree Star). Negative controls were obtained with exosome-coupled beads incubated with the secondary antibody. Sumoylation inhibition Cells were cultured with AA (100 μM) (Sigma) or DMSO for 4 h at 37 °C. Cells were then diluted 1:4 and incubated overnight. Exosomes and cells were resuspended in buffer 1 for western blotting or hnRNPA2B1 immunoprecipitation. Statistical analysis All statistical analyses were performed with Prism GraphPad. Statistical significance was calculated by nonparametric two-tailed Student’s t -test. When making multiple statistical comparisons on a single data set one-way ANOVA was used. Accession codes: The microarray analysis of activation-induced changes in the miRNA and mRNA profiles of primary T lymphoblasts and their exosomes has been uploaded to the NCBI Gene Expression Omnibus under GEO Series accession number GSE50972 . Proteomic raw data have been uploaded at Proteome Xchange under accession number PXD000350. How to cite this article: Villarroya-Beltri, C. et al. Sumoylated hnRNPAs2B1 controls the sorting of miRNAs into exosomes through binding to specific motifs. Nat. Commun. 4:2980 doi: 10.1038/ncomms3980 (2013).